A mouse model of adult-onset anaemia due to erythropoietin deficiency Erythropoietin regulates erythropoiesis in a hypoxia-inducible manner. Here we generate inherited super-anaemic mice (ISAM) as a mouse model of adult-onset anaemia caused by erythropoietin deficiency. ISAM express erythropoietin in the liver but lack erythropoietin production in the kidney. Around weaning age, when the major erythropoietin-producing organ switches from the liver to the kidney, ISAM develop anaemia due to erythropoietin deficiency, which is curable by administration of recombinant erythropoietin. In ISAM severe chronic anaemia enhances transgenic green fluorescent protein and Cre expression driven by the complete erythropoietin -gene regulatory regions, which facilitates efficient labelling of renal erythropoietin-producing cells. We show that the majority of cortical and outer medullary fibroblasts have the innate potential to produce erythropoietin, and also reveal a new set of erythropoietin target genes. ISAM are a useful tool for the evaluation of erythropoiesis-stimulating agents and to trace the dynamics of erythropoietin-producing cells. Red blood cell (RBC) production is finely controlled by erythropoietin (Epo) to maintain tissue oxygen homoeostasis [1] . Epo binds to its receptor (EpoR) on the erythroid precursors and induces downstream target genes to promote differentiation, proliferation and anti-apoptotic processes [2] . During mammalian development, the major Epo-producing organ shifts from the liver to the kidney along with the transition of haematopoietic tissues [3] , [4] , [5] . In the fetus, the hepatocyte-produced Epo supports fetal liver erythropoiesis via paracrine signalling [5] . Around birth, when the site of erythropoiesis changes to the bone marrow, renal Epo-producing (REP) cells in the peritubular interstitium of the kidney begin to secrete Epo [6] . Blood loss or reduced oxygen levels enhances renal and hepatic Epo secretion to induce stress erythropoiesis for normalizing the tissue oxygen supply [7] , [8] . The tissue-specific and hypoxia/anaemia-inducible production of Epo is stringently regulated at the gene transcriptional level. In the liver, Epo gene expression is activated by hypoxia-inducible transcription factors through its specific binding to the hypoxia-responsive element located 3′ to the Epo gene [9] , [10] , [11] . Using the bacterial artificial chromosome (BAC)-based transgenic mouse system, we recently demonstrated that the Epo gene 3′ enhancer (EpoE-3′) is necessary and sufficient for hypoxia-inducible transcription of the gene in hepatocytes [5] . Conversely, EpoE-3′ is dispensable for the regulation of kidney Epo expression, which appears to be controlled by distinct regulatory elements [12] , [13] . In addition, our transgenic mouse studies revealed that the GATA sequence located 30-base-pairs upstream from the transcription initiation site is essential for the constitutive suppression of ectopic Epo gene expression in other cells/tissues [14] . In kidneys, Epo expression is confined to specific fibroblastic cells, REP cells, predominantly located in the interstitial space of the corticomedullary junction [14] , [15] , [16] , [17] . While specific markers of REP cells have yet to be identified, we have developed a GFP (green fluorescent protein) reporter system for specific labelling of REP cells by means of targeted knock-in of GFP into the Epo gene locus. This system has demonstrated that REP cells possess a neural phenotype and connect with each other by their projections alongside renal tubules and vessels [6] , [14] , [17] . However, the nature of REP cells and molecular basis for Epo gene regulation within the cells are largely unknown. This is partly because the limited efficiency of identifying REP cells, as the number of Epo-expressing cells is transiently increased by the severity of the anaemic/hypoxic stress challenge experienced by the animals [14] , [18] , [19] . Furthermore, it remains unclear whether the Epo-producing potential or REP cell character is found in all renal interstitial cells or restricted to subpopulations of these cells. Renal or Epo-deficiency anaemia is often caused by insufficient Epo production in chronic kidney disease [20] . Recombinant Epo has been widely used to treat renal anaemia for more than 20 years, and next-generation erythropoiesis-stimulating agents (ESAs) have been developed [21] , [22] . As proper experimental animal systems of renal anaemia are still lacking, molecular effects and downstream target genes of recombinant Epo or ESAs in adult erythropoiesis have not been fully understood. Null mutations of either the Epo or EpoR gene cause embryonic lethal anaemia around day 12.5 (E12.5) in mice, clearly demonstrating the significance of Epo-EpoR signalling for fetal erythropoiesis [23] , [24] . In addition, conditional inactivation of either the Epo or Hif2α genes results in moderate anaemia (20–30% reduction in RBC numbers) in adult mice, suggesting the significance of Epo for adult erythropoiesis [25] , [26] . None of these mutants, however, represent good models of renal/Epo-deficiency anaemia. We recently generated homozygous EpoE-3′-deleted mice and discovered that the mice specifically lacked hepatic Epo expression after E14.5 and manifested severe anaemia in the perinatal period [5] . The mice, however, maintained normal adult erythropoiesis sufficiently supported by renal Epo production. This finding prompted us to develop a mouse model of Epo-deficiency anaemia by employing the transgenic complementation rescue technique for investigating regulation and function of Epo in adults. In this study, the Epo -null mutant mice are rescued from embryonic lethal anaemia by introducing an Epo transgene under the control of the GATA site and hepatic enhancer EpoE-3′. Supporting our hypothesis that the rescued mice would postnatally display Epo-deficiency anaemia without renal Epo expression, one transgene-rescued line presents severe adult-onset anaemia (60% RBC reduction) with undetectable levels of circulating Epo. We refer to this line of mice as ISAM (inherited super-anaemic mouse/mice). Our analyses of ISAM kidneys demonstrate that nearly all peritubular fibroblasts in the renal cortex and outer medulla have the potential to produce Epo as REP cells. The analyses of ISAM further delineate the functional roles of Epo in adult erythropoiesis. Epo transgene rescues Epo-null mice from embryonic lethality To attain liver-specific Epo expression, we constructed a 3.3 K-Epo3 ′ transgene based on the mouse Epo gene, which consisted of an 8.0-kilobase (kb) Epo gene fragment with a 0.3-kb sequence deletion in the 3′-untranslated region ( Fig. 1a , Tg ). 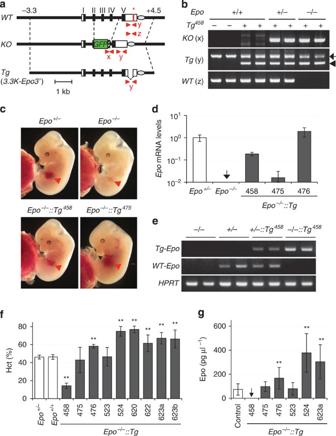Figure 1: Transgenic rescue ofEpoknockout mouse by3.3 K-Epo3′ transgene. (a) Structure of the wild-type (WT) and knockout (KO) alleles of theEpogene and3.3 K-Epo3′ transgene (Tg). In theKOallele, exons II–IV are replaced withGFPcDNA.Tgspans from 3.3-kb upstream to 4.5-kb downstream from the transcriptional start site, including the liver-specific enhancer EpoE-3′ (grey circle) with a 0.3-kb deletion in exon V. The open and solid boxes indicate untranslated and translated regions, respectively. (b) Representative data on genotyping PCR of offspring from transgenic rescue experiments using tail DNA (line-458). Positions of primer pairs (x, y and z) are indicated ina. The C57BL/6-specific sequence (asterisk ina) was detected with a primer pair z to distinguish theWTallele (C57BL/6) fromKOallele andTg(both are derived from the 129/Sv genome). (c) The liver (arrowheads) of theEpo–/–embryo is pale, whereas livers of rescued embryos (lines 458 and 475) are as red as theEpo+/–liver at E12.5. (d)EpomRNA levels in the E12.5 fetal liver.EpomRNA was expressed in the livers of rescued embryos (solid bars, lines 458, 475 and 476), but not detected in theEpo–/–liver (arrow indicates undetectable levels). Data represent relative expression levels when the level of littermateEpo+/–liver is set as 1 (means±s.d.,n=3–7). (e) Expressions ofTgand endogenousEpomRNA were detected separately by semi-quantitative RT–PCR analysis. E12.5 fetal livers from line-458 littermate embryos were analysed.HPRTwas used as an internal control. (f) Hct of the rescued (solid bars) and control mice (open bars) at 8–14 weeks of age. Data are the means±s.d. (n=4–37). **P<0.005 compared withEpo+/+mice (Student’st-test). (g) Plasma Epo concentrations of the rescued (solid bars) and control (open bar,Epo+/+andEpo+/–) mice at 8–29 weeks of age. Data are the means±s.d. (n=6–22). **P<0.005 compared with control mice (Student’st-test). With this construct, we established eleven transgenic mouse lines with a variety of transgene copy numbers ( Table 1 ). These Tg mice were crossed with Epo +/– mice harbouring an Epo knock-in/knockout allele in which the Epo-coding region was replaced with GFP complementary DNA (cDNA) [6] ( Fig. 1a, KO ). We found that the Epo transgene rescued the Epo –/– mice from embryonic lethality in nine transgenic lines ( Fig. 1b and Table 1 ). Epo –/– embryos suffered from severe anaemia and died around E12.5, consistent with previous reports [23] , [25] . In contrast, the transgene sustained fetal liver erythropoiesis and rescued the Epo –/– embryos from the lethal anaemia ( Fig. 1c ). Figure 1: Transgenic rescue of Epo knockout mouse by 3.3 K - Epo3 ′ transgene. ( a ) Structure of the wild-type ( WT ) and knockout ( KO ) alleles of the Epo gene and 3.3 K - Epo3 ′ transgene ( Tg ). In the KO allele, exons II–IV are replaced with GFP cDNA. Tg spans from 3.3-kb upstream to 4.5-kb downstream from the transcriptional start site, including the liver-specific enhancer EpoE-3′ (grey circle) with a 0.3-kb deletion in exon V. The open and solid boxes indicate untranslated and translated regions, respectively. ( b ) Representative data on genotyping PCR of offspring from transgenic rescue experiments using tail DNA (line-458). Positions of primer pairs (x, y and z) are indicated in a . The C57BL/6-specific sequence (asterisk in a ) was detected with a primer pair z to distinguish the WT allele (C57BL/6) from KO allele and Tg (both are derived from the 129/Sv genome). ( c ) The liver (arrowheads) of the Epo –/– embryo is pale, whereas livers of rescued embryos (lines 458 and 475) are as red as the Epo +/– liver at E12.5. ( d ) Epo mRNA levels in the E12.5 fetal liver. Epo mRNA was expressed in the livers of rescued embryos (solid bars, lines 458, 475 and 476), but not detected in the Epo –/– liver (arrow indicates undetectable levels). Data represent relative expression levels when the level of littermate Epo +/– liver is set as 1 (means±s.d., n =3–7). ( e ) Expressions of Tg and endogenous Epo mRNA were detected separately by semi-quantitative RT–PCR analysis. E12.5 fetal livers from line-458 littermate embryos were analysed. HPRT was used as an internal control. ( f ) Hct of the rescued (solid bars) and control mice (open bars) at 8–14 weeks of age. Data are the means±s.d. ( n =4–37). ** P <0.005 compared with Epo +/+ mice (Student’s t -test). ( g ) Plasma Epo concentrations of the rescued (solid bars) and control (open bar, Epo +/+ and Epo +/– ) mice at 8–29 weeks of age. Data are the means±s.d. ( n =6–22). ** P <0.005 compared with control mice (Student’s t -test). Full size image Table 1 Number of Epo −/− ::Tg pups from Epo +/− ::Tg and Epo +/− parents. Full size table Epo messenger RNA (mRNA) expression was detected in the E12.5 fetal livers of the rescued embryos but not in the Epo –/– fetal livers ( Fig. 1d ). We confirmed that the Epo mRNA in the rescued embryos originated from the transgene using specific primer sets ( Fig. 1e ). The transgene expression of the rescued embryos was higher than that of Epo +/– ::Tg embryos, suggesting inducible regulation of the transgene in the fetal liver. In addition, anaemic stress increased transgene expression in the adult liver of the rescued mice, whereas the transgene expression level was almost unchanged in other organs ( Supplementary Fig. S1a ). These results indicate the functional sufficiency of the regulatory regions within the 3.3 K-Epo3 ′ transgene for hypoxia/anaemia-inducible expression of the Epo gene in fetal and adult livers. While the Epo mRNA expression level was comparable between Epo –/– ::Tg 476 and Epo +/– livers, the mRNA levels in Epo –/– ::Tg 458 and Epo –/– ::Tg 475 livers were lower than those in the Epo +/– liver (~20% and 2%, respectively; Fig. 1d ). As these rescued embryos maintained fetal liver erythropoiesis ( Fig. 1c ), this finding suggested that ectopic transgene expression might support the erythropoiesis ( Supplementary Fig. S1b ). Indeed, we found constitutive and ectopic transgene expressions in various organs of the adult rescued mice ( Supplementary Fig. S1a ). The hyper-produced Epo provoked polycythaemia in six rescued lines ( Fig. 1f ). The polycythaemic mice showed high Epo concentrations in the plasma compared with the control mice ( Fig. 1g ), indicating that the employed regulatory regions are insufficient for suppression of the integration-position effect of the transgene expression. A Tg -rescued line with adult-onset Epo-deficiency anaemia We noticed that the line-458 rescued mice ( Epo –/– ::Tg 458 ) suffered from severe anaemia ( Fig. 2a ) with markedly lower haematocrit (Hct) than the other lines ( Fig. 1f ). The rescued mice showed no apparent abnormality in embryonic erythropoiesis ( Fig. 1c ). Surprisingly, circulating Epo was nearly undetectable in the plasma ( Fig. 1g ). Therefore, we carried out further characterization of the Epo –/– ::Tg 458 mice, or ISAM, as a new animal model for Epo-deficiency anaemia. 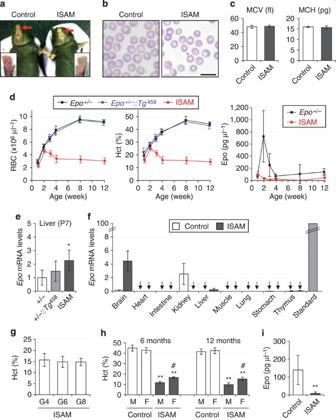Figure 2: Severe adult-onset anaemia with Epo-deficiency inEpo–/–::Tg458mice. (a) The snout (arrow) and paws (inlet) ofEpo–/–::Tg458mice (ISAM) are whiter than those of controlEpo+/–mice. (b) Wright-Giemsa staining of peripheral blood smears from ISAM and control mice. Scale bar, 20 μm. (c) MCV (mean corpuscular volume) and MCH (mean corpuscular haemoglobin) values in ISAM (n=26) and control mice (n=13) at 8 weeks of age. Data are the means±s.d. (d) RBC counts, Hct and plasma Epo concentrations of ISAM and littermate control mice (Epo+/–andEpo+/–::Tg458) are monitored up to 12 weeks of age. Data are the means±s.d. (n=7–21). (e)EpomRNA levels in the liver of indicated genotype mice at postnatal day 7 (P7). Data are the means±s.d. (n=4–6). *P<0.05 compared withEpo+/–mice (Student’st-test). (f)EpomRNA levels in the indicated organs from ISAM (solid bar) and controlEpo+/–mice (open bar) at 12 weeks of age. Data represent relative expression levels when the level of a standard sample (kidneys of anaemicEpo+/–mice, grey bar) is set as 100 (means±s.d.,n=3). Arrows indicate undetectable expression levels. (g) Hct of ISAM at 8–14 weeks of age was compared in the 4th, 6th and 8th generations (G4, G6 and G8, respectively) from the transgenic founder. Data are the means±s.d. (n=6–11). (h) Hct of ISAM (solid bar) and control mice (Epo+/–andEpo+/–::Tg458, open bar) at 6 and 12 months of age. Hct of female (F) ISAM is higher than that of male (M) ISAM (#P<0.05 by Student’st-test). Data are the means±s.d. (n=5–23). **P<0.005 compared with age- and sex-matched control mice (Student’st-test). (i) Plasma Epo concentrations in ISAM (n=21) and control mice (n=6) at 12 months of age. Data are the means±s.d. **P<0.005 compared with control mice (Student’st-test). Figure 2: Severe adult-onset anaemia with Epo-deficiency in Epo –/– ::Tg 458 mice. ( a ) The snout (arrow) and paws (inlet) of Epo –/– ::Tg 458 mice (ISAM) are whiter than those of control Epo +/– mice. ( b ) Wright-Giemsa staining of peripheral blood smears from ISAM and control mice. Scale bar, 20 μm. ( c ) MCV (mean corpuscular volume) and MCH (mean corpuscular haemoglobin) values in ISAM ( n =26) and control mice ( n =13) at 8 weeks of age. Data are the means±s.d. ( d ) RBC counts, Hct and plasma Epo concentrations of ISAM and littermate control mice ( Epo +/– and Epo +/– ::Tg 458 ) are monitored up to 12 weeks of age. Data are the means±s.d. ( n =7–21). ( e ) Epo mRNA levels in the liver of indicated genotype mice at postnatal day 7 (P7). Data are the means±s.d. ( n =4–6). * P <0.05 compared with Epo +/– mice (Student’s t -test). ( f ) Epo mRNA levels in the indicated organs from ISAM (solid bar) and control Epo +/– mice (open bar) at 12 weeks of age. Data represent relative expression levels when the level of a standard sample (kidneys of anaemic Epo +/– mice, grey bar) is set as 100 (means±s.d., n =3). Arrows indicate undetectable expression levels. ( g ) Hct of ISAM at 8–14 weeks of age was compared in the 4th, 6th and 8th generations (G4, G6 and G8, respectively) from the transgenic founder. Data are the means±s.d. ( n =6–11). ( h ) Hct of ISAM (solid bar) and control mice ( Epo +/– and Epo +/– ::Tg 458 , open bar) at 6 and 12 months of age. Hct of female (F) ISAM is higher than that of male (M) ISAM (# P <0.05 by Student’s t -test). Data are the means±s.d. ( n =5–23). ** P <0.005 compared with age- and sex-matched control mice (Student’s t -test). ( i ) Plasma Epo concentrations in ISAM ( n =21) and control mice ( n =6) at 12 months of age. Data are the means±s.d. ** P <0.005 compared with control mice (Student’s t -test). Full size image In the peripheral blood of ISAM, the morphology, size and haemoglobin content of erythrocytes were comparable with those of normal mice ( Fig. 2b ). White blood cell and platelet counts were also within the normal range ( Supplementary Fig. S2a ). Despite the profound anaemia, reticulocytes were maintained at low levels ( Supplementary Fig. S2b ). These phenotypes were consistent with normochromic/normocytic anaemia with hypo-proliferation of erythrocyte precursors caused by Epo-insufficiency [20] . After birth, normal mice showed an increase of RBC and Hct levels along with their growth that reached constant levels by 8 weeks ( Fig. 2d ). In contrast, while ISAM showed a RBC increase up to 2 weeks of age, they developed anaemia thereafter. The body weight increase of ISAM was normal ( Supplementary Fig. S2c ). Plasma Epo concentrations of ISAM diminished to almost undetectable levels from 2 weeks after birth, whereas those of control mice transiently increased during erythroid expansion ( Fig. 2d ). The possibility that the transgene insertion caused the anaemia in ISAM was excluded, because Epo +/– ::Tg 458 mice showed normal erythropoietic activities. ISAM fail to switch Epo production from liver to kidney We investigated switching of Epo-producing organs from the perinatal liver to the adult kidney in ISAM. At postnatal day 7 (P7), the Epo mRNA level in ISAM livers was higher than that of the control livers ( Fig. 2e ). We detected Epo mRNA expression in normal mouse kidneys at P7 but not in ISAM kidneys ( Supplementary Fig. S2d ). In adult control mice, Epo mRNA expression was specifically detected in the kidney, whereas it was undetected in the liver ( Fig. 2f ). On the contrary, Epo mRNA was detected in the liver but not in the kidney of adult ISAM, suggesting that anaemia induced the liver-specific transgene expression. Indeed, Epo mRNA expression decreased to undetectable levels in the ISAM liver after recovery from anaemia by recombinant human EPO (rHuEPO) treatment ( Supplementary Fig. S2e ). However, the hepatic Epo expression appeared to be insufficient to sustain erythropoiesis in ISAM. We observed that the brain of ISAM constitutively expressed Epo mRNA at a level ~18-fold higher than that of the liver ( Fig. 2f and Supplementary Fig. S2e ). It is possible that the brain-produced Epo failed to contribute to the circulation owing to the blood–brain barrier [7] , [8] , [27] . Taken together, Epo -null mice are fully rescued from lethality by 3.3 K-Epo3 ′ transgene expression in the perinatal liver, but ISAM develops adult-onset Epo-deficiency anaemia due to the failure of renal Epo production and compensatory Epo secretion from extra-renal tissues. Genetically reproducible chronic anaemia of ISAM ISAM were born at an expected ratio in several interbreeding experiments ( Table 2 ). The anaemic phenotype was well reproduced in subsequent mouse generations ( Fig. 2g ). From intercrossing of ISAM parents, we obtained ISAM with a homozygous transgene phenotype ( Epo –/– ::Tg 458/458 ), which also suffered from severe Epo-deficient anaemia without apparent abnormalities in fertility ( Table 2 and Supplementary Fig. S2f ). The life span was more than 1 year in most ISAM, while serious anaemia was continuously observed at 6 and 12 months of age ( Fig. 2h ). Table 2 Number of pups from ISAM parents. Full size table The anaemia in ISAM was slightly more severe in males than in females, as well as in aged mice than in young mice ( Fig. 2h ). The plasma Epo level was nearly undetectable in 12-month-old ISAM, suggesting sustained Epo-deficiency throughout adulthood ( Fig. 2i ). We found that cardiomegaly was elicited in ISAM ( Supplementary Fig. S3a,b ) to compensate for the anaemia with increased cardiac output [28] . These results indicate that ISAM represents a valuable resource as a genetically reproducible animal model for severe chronic anaemia. Erythropoietic defects caused by insufficient Epo production In ISAM, the distal femur was pale ( Fig. 3a ), while the bone marrow histology was apparently normal ( Fig. 3b ). Cells in the bone marrow were significantly decreased compared with control mice ( Fig. 3c ). We also analysed spleen, the erythropoietic organ more responsible than bone marrow for stress erythropoiesis in rodents [29] , [30] . In control mice, phlebotomy-induced anaemia enlarged the spleen for compensatory stress erythropoiesis, but the size and weight of the spleen remained largely normal in ISAM regardless of severe anaemia ( Fig. 3a and Supplementary Fig. S3c ). Total splenic cells were reduced in ISAM without any changes of splenic architecture ( Fig. 3b ). 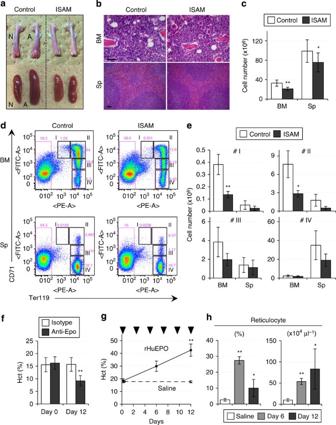Figure 3: Erythroblast-specific defects caused by insufficient Epo production in ISAM. (a) Macroscopic appearance of femurs (upper) and spleen (lower) from ISAM and control mice (Epo+/–) under normal (N) or acute anaemic (A) conditions at 12 weeks of age. (b) Representative haematoxylin and eosin staining of bone marrow (BM) and spleen (Sp) sections from ISAM and control mice. Scale bars, 100 μm. (c) Total cell numbers in BM (per femur) and Sp from ISAM and control mice (Epo+/–andEpo+/–::Tg458) at 8–12 weeks of age. Data are the means±s.d. (n=8–10). (d) Representative data of flow cytometry of CD71 and Ter119 expressions in bone marrow (BM) and spleen (Sp) from ISAM and control mice at 12 weeks of age. (e) Cell numbers in each erythroid fraction (I–IV ind) are shown as the means±s.d. (n=3–5). Similar results were obtained in an independent experiment (n=5). (f) Hct of ISAM at 7–8 weeks of age before (day 0) and after (day 12) intraperitoneal injection of neutralizing anti-Epo antibody every other day. Isotype antibody was injected in a control group. Data are the means±s.d. (n=6). (g) Hct of ISAM at 11–15 weeks of age before (day 0) and after (days 6 and 12) injected rHuEPO (3,000 U kg–1body weight) or saline every other day (arrowhead). Data are the means±s.d. (n=4). (h) Percentages and counts of reticulocytes on day 6 and 12 as ing. Data from saline-injected ISAM on day 12 were used as a control. Data are the means±s.d. (n=4). *P<0.05, **P<0.005 compared with control samples by Student’st-test (c,e–h). Figure 3: Erythroblast-specific defects caused by insufficient Epo production in ISAM. ( a ) Macroscopic appearance of femurs (upper) and spleen (lower) from ISAM and control mice ( Epo +/– ) under normal (N) or acute anaemic (A) conditions at 12 weeks of age. ( b ) Representative haematoxylin and eosin staining of bone marrow (BM) and spleen (Sp) sections from ISAM and control mice. Scale bars, 100 μm. ( c ) Total cell numbers in BM (per femur) and Sp from ISAM and control mice ( Epo +/– and Epo +/– ::Tg 458 ) at 8–12 weeks of age. Data are the means±s.d. ( n =8–10). ( d ) Representative data of flow cytometry of CD71 and Ter119 expressions in bone marrow (BM) and spleen (Sp) from ISAM and control mice at 12 weeks of age. ( e ) Cell numbers in each erythroid fraction (I–IV in d ) are shown as the means±s.d. ( n =3–5). Similar results were obtained in an independent experiment ( n =5). ( f ) Hct of ISAM at 7–8 weeks of age before (day 0) and after (day 12) intraperitoneal injection of neutralizing anti-Epo antibody every other day. Isotype antibody was injected in a control group. Data are the means±s.d. ( n =6). ( g ) Hct of ISAM at 11–15 weeks of age before (day 0) and after (days 6 and 12) injected rHuEPO (3,000 U kg –1 body weight) or saline every other day (arrowhead). Data are the means±s.d. ( n =4). ( h ) Percentages and counts of reticulocytes on day 6 and 12 as in g . Data from saline-injected ISAM on day 12 were used as a control. Data are the means±s.d. ( n =4). * P <0.05, ** P <0.005 compared with control samples by Student’s t -test ( c , e – h ). Full size image Using flow cytometry, we examined erythrocyte maturation separated into four erythroblastic fractions (I–IV) with expressions of cell surface antigens, CD71 (transferrin receptor) and Ter119 (refs 31 , 32 ). The number of cells in fractions I (CD71 high Ter119 low , proerythroblasts) and II (CD71 high Ter119 high , basophilic erythroblasts) was strikingly decreased in the bone marrow of ISAM ( Fig. 3d ). These early erythroblasts also tended to decrease in the spleen of ISAM. The CD71 high Ter119 – c-Kit + fraction, including erythroid progenitors [32] , was unaffected in the bone marrow and spleen of ISAM ( Supplementary Fig. S4a,b ). These data are consistent with previous reports showing that Epo-deficiency reduces erythroblasts without changes in differentiation and proliferation of the erythroid progenitors in the embryonic and neonatal stages [5] , [23] , [33] . Intraperitoneal injection of an Epo-neutralizing antibody further decreased the Hct of ISAM ( Fig. 3f ), demonstrating that the minimal level of circulating Epo was able to support erythropoiesis for the survival of ISAM. Conversely, administration of rHuEPO every other day for 12 days restored the Hct to normal levels with a significant increase in reticulocytes ( Fig. 3g ), indicating that stress erythropoiesis is provoked in ISAM by Epo-treatment. These data unequivocally demonstrate that the anaemic phenotype of ISAM is caused by Epo-insufficiency and that ISAM is suitable for in vivo assessments of ESAs for Epo-dependent anaemia. Identification of Epo-responsive haematopoietic genes in vivo To identify Epo-regulated genes using the Epo-deficient condition of ISAM, we analysed mRNA expression profile in haematopoietic cells. A microarray analysis was conducted using RNA samples prepared from the bone marrow of ISAM 6 h after rHuEPO injection. We found that the expression of ~400 genes was significantly changed more than 1.5-fold by Epo stimulation, of which 202 genes were upregulated and 192 genes were downregulated ( Fig. 4a and Supplementary Data ). rHuEpo administration increased the expression of genes related to membrane cytoskeletons, transporters, glycolytic enzymes and transcription factors, which have key roles in erythroid differentiation. The upregulated group contained Cish , Gdf3 , Pim1 , Tfrc , Egr1 and Podxl genes, which were known as Epo-responsive erythroid genes [34] , [35] (circles in Fig. 4a ). In contrast, Epo stimulation repressed expression of genes related to cell adhesion ( Itga4 ) ( [36] , [37] ) and extracellular matrix remodelling. 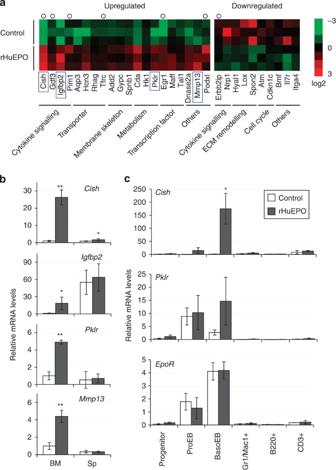Figure 4: Identification of Epo-responsive haematopoietic genes using ISAM. (a) Heat map data depicting mRNA expression changes in the bone marrow (BM) of ISAM 6 h after rHuEPO injection (3,000 U kg–1body weight). Thirty representative genes, expression levels of which were significantly changed >1.5-fold between the rHuEPO and control groups (P<0.05 by Student’st-test,n=3 for each), are listed with their functional categories. ECM, extracellular matrix. Circles indicate genes previously reported as Epo-responsive erythroid genes. Genome-wide data from the microarray analysis are available online (see Methods). PBS-injected or non-treated ISAM was used as a control group. (b) RT–qPCR analysis ofCish,Igfbp2,PklrandMmp13mRNA levels (highlighted with blue boxes ina) in the BM and spleen (Sp) from ISAM 6 h after rHuEPO injection. Data represent relative expression levels when the levels of control BM are set as 1 (means±s.d.,n=3–5). *P<0.05, **P<0.005 compared with control samples (Student’st-test). (c) BM cells of ISAM 6 h after rHuEPO or PBS (Control) injection were fractionated into CD71highTer119–c-Kit+(progenitor), CD71highTer119low(ProEB), CD71highTer119high(BasoEB), Gr1+and Mac1+(Gr1/Mac1+), B220+and CD3+populations. RT–qPCR analysis ofCish,PklrandEpoRmRNA levels in the cell fraction of BM from ISAM 6 h after rHuEPO or PBS (Control) injection. Data represent relative expression levels when the levels of BM from untreated ISAM are set as 1 (means±s.d.,n=3). *P<0.05 compared with control samples (Student’st-test). Figure 4: Identification of Epo-responsive haematopoietic genes using ISAM. ( a ) Heat map data depicting mRNA expression changes in the bone marrow (BM) of ISAM 6 h after rHuEPO injection (3,000 U kg –1 body weight). Thirty representative genes, expression levels of which were significantly changed >1.5-fold between the rHuEPO and control groups ( P <0.05 by Student’s t -test, n =3 for each), are listed with their functional categories. ECM, extracellular matrix. Circles indicate genes previously reported as Epo-responsive erythroid genes. Genome-wide data from the microarray analysis are available online (see Methods). PBS-injected or non-treated ISAM was used as a control group. ( b ) RT–qPCR analysis of Cish , Igfbp2 , Pklr and Mmp13 mRNA levels (highlighted with blue boxes in a ) in the BM and spleen (Sp) from ISAM 6 h after rHuEPO injection. Data represent relative expression levels when the levels of control BM are set as 1 (means±s.d., n =3–5). * P <0.05, ** P <0.005 compared with control samples (Student’s t -test). ( c ) BM cells of ISAM 6 h after rHuEPO or PBS (Control) injection were fractionated into CD71 high Ter119 – c-Kit + (progenitor), CD71 high Ter119 low (ProEB), CD71 high Ter119 high (BasoEB), Gr1 + and Mac1 + (Gr1/Mac1 + ), B220 + and CD3 + populations. RT–qPCR analysis of Cish , Pklr and EpoR mRNA levels in the cell fraction of BM from ISAM 6 h after rHuEPO or PBS (Control) injection. Data represent relative expression levels when the levels of BM from untreated ISAM are set as 1 (means±s.d., n =3). * P <0.05 compared with control samples (Student’s t -test). Full size image The microarray data provided a novel finding that Igfbp2 , Pklr and Mmp13 genes were activated by Epo signalling (blue boxes in Fig. 4a ). The induction of these genes was confirmed in the bone marrow by quantitative reverse transcription PCR (RT–qPCR) analyses ( Fig. 4b ). These changes were not significant in the spleen, possibly reflecting the differences in Epo-sensitivity or cellular populations between these organs. The changes of Hk1 , Spon2 , Cdkn1c, Itga4 and Bmf expression levels were also validated by RT–qPCR ( Supplementary Fig. S5 ). To determine the cell fraction that responded to Epo stimulation among haematopoietic cells, we conducted RT–qPCR in fractionated bone marrow cells from ISAM with or without Epo administration. Cish, Pklr and Hk1 mRNA expressions were induced by Epo stimulation in erythroblast fractions, in which EpoR mRNA level is exclusively high regardless of Epo administration ( Fig. 4c and Supplementary Fig. S6 ). These data indicate that Epo signalling directly upregulates expressions of Cish, Pklr and Hk1 genes in the erythroblastic cells. Igfbp2 and Mmp13 genes were reported to be predominantly expressed in stromal cells and osteoblasts [38] , [39] . We confirmed that these genes were highly expressed in primary mouse osteoblasts compared with the bone marrow, while the expression levels were unchanged by rHuEPO ( Supplementary Fig. S7 ). As EpoR mRNA expression was very weak in osteoblasts ( Supplementary Fig. S7 ), we surmise that Epo administration activates the Igfbp2 and Mmp13 gene expressions in the ISAM bone marrow through indirect mechanisms and that Epo-stimulated erythroblasts affect the bone marrow microenvironment [34] , [40] . Chronic anaemia induces GFP expression from the Epo KO allele As GFP cDNA is knocked-in to the Epo gene, the KO allele expresses GFP instead of Epo under the hypoxia-inducible regulatory system. We hypothesized that chronic anaemia in ISAM would induce enhanced GFP expression and this would offer efficient detection of REP cells. The GFP mRNA expression level was significantly higher in ISAM than in Epo +/– mice bearing the GFP -knock-in allele heterozygously ( Fig. 5a ). The highest GFP mRNA expression in ISAM was detected in the kidney, while the second highest expression was in the liver, correlating with the endogenous Epo expression profile [14] . The anaemia-inducibility of GFP mRNA expression was verified as its expression was markedly diminished when anaemia was reversed by rHuEPO ( Supplementary Fig. S8 ). 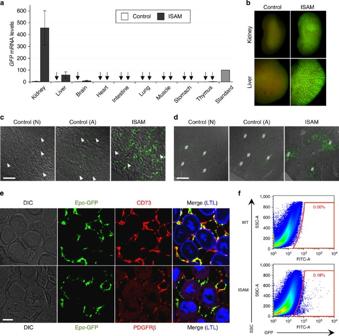Figure 5: Severe chronic anaemia of ISAM leads to efficient labelling of REP cells with GFP. (a)GFPmRNA levels in the indicated organs from ISAM (solid bars) and controlEpo+/–mice (open bars) at 12 weeks of age. Data represent relative expression levels when the level of the standard sample (kidneys of anaemicEpo+/–mice, grey bar) is set as 100 (means±s.d.,n=3). Arrows indicate undetectable expression levels. (b) GFP expression in the kidney and liver from ISAM and controlEpo+/–mice. (c, d) Distribution of GFP-labelled Epo-producing cells in the kidney cortex (c) and liver (d) of ISAM and controlEpo+/–mice under normal (N) and acute anaemic (A) conditions. In the ISAM kidney, GFP-labelled REP cells were broadly identified from the deep (top sides in the panels) to the subcapsular (bottom sides) cortex (arrowheads, glomeruli). In the ISAM liver, many hepatocytes surrounding the central veins (#) expressed GFP. (e) Immunohistochemical analyses of GFP-labelled REP cells in the ISAM kidney. GFP-labelled REP cells (green) expressed CD73 (red, upper) and PDGFRβ (red, lower) in the interstitial space among renal tubules.Lotus TetragonolobusLectin (LTL, blue) was used to stain the proximal tubules. DIC, differential interference contrast microscope; Scale bars, 200 μm (c,d) and 20 μm (e). (f) Flow cytometry of GFP expression in the single-cell suspension of the ISAM kidneys. The percentages of GFP-positive cells are shown (red region). SSC, side scatter. Figure 5: Severe chronic anaemia of ISAM leads to efficient labelling of REP cells with GFP. ( a ) GFP mRNA levels in the indicated organs from ISAM (solid bars) and control Epo +/– mice (open bars) at 12 weeks of age. Data represent relative expression levels when the level of the standard sample (kidneys of anaemic Epo +/– mice, grey bar) is set as 100 (means±s.d., n =3). Arrows indicate undetectable expression levels. ( b ) GFP expression in the kidney and liver from ISAM and control Epo +/– mice. ( c, d ) Distribution of GFP-labelled Epo-producing cells in the kidney cortex ( c ) and liver ( d ) of ISAM and control Epo +/– mice under normal (N) and acute anaemic (A) conditions. In the ISAM kidney, GFP-labelled REP cells were broadly identified from the deep (top sides in the panels) to the subcapsular (bottom sides) cortex (arrowheads, glomeruli). In the ISAM liver, many hepatocytes surrounding the central veins (#) expressed GFP. ( e ) Immunohistochemical analyses of GFP-labelled REP cells in the ISAM kidney. GFP-labelled REP cells (green) expressed CD73 (red, upper) and PDGFRβ (red, lower) in the interstitial space among renal tubules. Lotus Tetragonolobus Lectin (LTL, blue) was used to stain the proximal tubules. DIC, differential interference contrast microscope; Scale bars, 200 μm ( c , d ) and 20 μm ( e ). ( f ) Flow cytometry of GFP expression in the single-cell suspension of the ISAM kidneys. The percentages of GFP-positive cells are shown (red region). SSC, side scatter. Full size image GFP expression in the kidney and liver of ISAM was visible through the fluorescent microscope ( Fig. 5b ), which was attributable to the numerous Epo-producing cells expressing GFP ( Fig. 5c ). Notably, GFP-labelled REP cells were broadly distributed in the cortical and outer medullary interstitium of the ISAM kidney, while its distribution was limited to the deep cortex in the control mouse kidneys under acute anaemic conditions ( Fig. 5c ). The GFP-positive cells were located in the peritubular interstitial space and expressed CD73 and PDGFRβ ( Fig. 5e ), both of which are surface markers for renal fibroblasts including REP cells [6] , [15] , [16] , [41] , [42] . REP cells were also identified as a GFP-positive fraction from the renal cell suspension of adult ISAM using flow cytometry ( Fig. 5f ). Thus, ISAM facilitates the efficient monitoring of REP cells without any external stimuli. Epo-Cre combined with ISAM efficiently labels REP cells We further aimed to identify renal cells that possess the potential to produce Epo by using the Cre- lox P labelling system [43] . To express Cre recombinase in the Epo-expressing cells, we exploited the BAC transgenic mouse system using the 180-kb mouse Epo gene regulatory region, which is sufficient for Epo gene regulation in vivo [14] ( Epo-Cre , Fig. 6a ). Three Epo-Cre transgenic mouse lines were established (lines 44, 47 and 48) and mated with the reporter mouse line for Cre-mediated recombination ( Rosa26-STOP-tdTomato [44] , R26T in this study). In this mouse line, cells that once caused the recombination are continuously labelled with robust tdTomato (red fluorescent protein) expression. 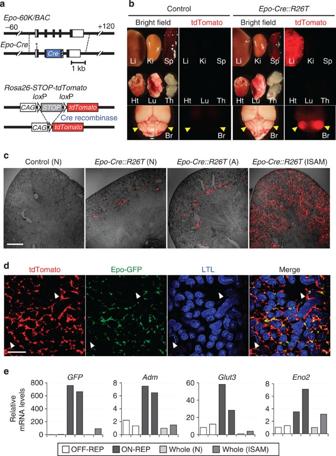Figure 6: Distribution of cells with Epo-producing potential throughout the renal cortex. (a) Structure ofEpo-Cretransgene (upper) and scheme of reporter system for Cre-mediate recombination inRosa26-STOP-tdTomatomouse (R26T, lower).CrecDNA was integrated into the mouse genomic BAC clone (Epo-60 K/BAC) containing 60-kb upstream and 120-kb downstream regions ofEpogene. The start codon in the exon I was mutated (asterisk) to use the start codon ofCrecDNA in theEpo-Cretransgene. After the Cre-mediated excision of theSTOPsequence betweenloxP sites in theR26Tallele, the cell initiates constitutive tdTomato expression driven by theCAGpromoter. (b) Expression of tdTomato fluorescence (red) inEpo-Cre::R26T(line 44) and controlR26Tmice. Li, liver; Ki, kidney; Sp, spleen; Ht, heart; Lu, lung; Th, thymus; Br, brain; arrowheads, cerebellum. (c) Distribution of tdTomato-positive cells in the kidney ofEpo-Cre::R26T(line 44) and control mice under normal (N) and acute anaemic (A) conditions. tdTomato expression was also tested in the ISAM genetic background. (d) Immunohistochemical analysis of tdTomato-positive cells in the kidney cortex of ISAM::Epo-Cre::R26Tcompound mice (line 44). GFP-labelled REP cells (green) overlapped with tdTomato-expressing cells (red). Most fibroblastic cells in the interstitial space among renal tubules stained byLotus TetragonolobusLectin (LTL) (blue) are positive for tdTomato expression. Arrowhead, glomeruli; Scale bars, 500 μm (c) and 100 μm (d). (e) RT–qPCR analysis ofGFP,Adm,Glut3andEno2mRNA levels in sorted OFF-REP (tdTomato+GFP–) and ON-REP (tdTomato+GFP+) cells isolated from the ISAM::Epo-Cre::R26Tkidneys (line 44) by flow cytometry. The expression levels were also examined in whole kidneys from ISAM and control mice (N). Data represent relative expression levels when the level of control kidney is set as 1 (n=2). Figure 6: Distribution of cells with Epo-producing potential throughout the renal cortex. ( a ) Structure of Epo-Cre transgene (upper) and scheme of reporter system for Cre-mediate recombination in Rosa26-STOP-tdTomato mouse ( R26T , lower). Cre cDNA was integrated into the mouse genomic BAC clone ( Epo-60 K/BAC ) containing 60-kb upstream and 120-kb downstream regions of Epo gene. The start codon in the exon I was mutated (asterisk) to use the start codon of Cre cDNA in the Epo-Cre transgene. After the Cre-mediated excision of the STOP sequence between lox P sites in the R26T allele, the cell initiates constitutive tdTomato expression driven by the CAG promoter. ( b ) Expression of tdTomato fluorescence (red) in Epo-Cre::R26T (line 44) and control R26T mice. Li, liver; Ki, kidney; Sp, spleen; Ht, heart; Lu, lung; Th, thymus; Br, brain; arrowheads, cerebellum. ( c ) Distribution of tdTomato-positive cells in the kidney of Epo-Cre::R26T (line 44) and control mice under normal (N) and acute anaemic (A) conditions. tdTomato expression was also tested in the ISAM genetic background. ( d ) Immunohistochemical analysis of tdTomato-positive cells in the kidney cortex of ISAM:: Epo-Cre::R26T compound mice (line 44). GFP-labelled REP cells (green) overlapped with tdTomato-expressing cells (red). Most fibroblastic cells in the interstitial space among renal tubules stained by Lotus Tetragonolobus Lectin (LTL) (blue) are positive for tdTomato expression. Arrowhead, glomeruli; Scale bars, 500 μm ( c ) and 100 μm ( d ). ( e ) RT–qPCR analysis of GFP , Adm , Glut3 and Eno2 mRNA levels in sorted OFF-REP (tdTomato + GFP – ) and ON-REP (tdTomato + GFP + ) cells isolated from the ISAM:: Epo-Cre::R26T kidneys (line 44) by flow cytometry. The expression levels were also examined in whole kidneys from ISAM and control mice (N). Data represent relative expression levels when the level of control kidney is set as 1 ( n =2). Full size image The tdTomato fluorescence was detected mainly in the liver and brain of Epo-Cre::R26T mice with different efficiencies of recombination ( Fig. 6b and Supplementary Fig. S9 ). As the basal Epo expression was very weak in the adult liver and brain, the tdTomato expressions most likely reflected the fate tracing of Epo-Cre recombination in hepatocytes and neural lineage cells in the embryonic stages (N.S., unpublished observation). In the Epo-Cre::R26T kidney, we observed tdTomato-positive cells in the peritubular interstitial space around the corticomedullary boundary under normal and acute anaemic conditions ( Fig. 6c and Supplementary Fig. S10 ). The tdTomato-positive cells were practically identical to REP cells as shown by the fibroblastic shape and CD73 expression ( Supplementary Fig. S11 ). Importantly, induction of the Epo-Cre recombination by severe chronic anaemia in ISAM led to a dramatic increase in the number of tdTomato-positive cells in kidneys, which were widely spread in the cortical and outer medullary interstitium ( Fig. 6c ). The number of tdTomato-labelled cells was greater than the number of GFP-labelled cells, suggesting that Epo-Cre recombination was induced in a large number of REP cells at random ( Fig. 6d ). As the anaemia in ISAM was initiated after kidney development, the recombination efficiency was comparable between ISAM and control background mice at 2 weeks of age ( Supplementary Fig. S12 ). These results indicate that terminally maturated cells activate the Epo-Cre transgene expression by their own Epo-producing ability in response to severe anaemia. Thus, potentially Epo-producing cells are broadly distributed in the cortical and outer medullary interstitium as peritubular fibroblasts. Flow cytometry analyses demonstrated that about 10% of tdTomato-positive cells were positive for GFP expression (‘ON-REP’, tdTomato + GFP + fraction) in kidneys of ISAM bearing Epo-Cre::R26T loci ( Supplementary Fig. S13a ). This result indicates that the Epo gene locus is inactive in the majority of REP cells (‘OFF-REP’, tdTomato + GFP – fraction). To elucidate expression profiles related to the inducible Epo gene transcription in REP cells, we compared expressions of hypoxia-inducible genes between ON-REP and OFF-REP fractions. We found that Adm , Glut3 and Eno2 genes [45] , [46] , [47] were strongly expressed in ON-REP cells compared with OFF-REP cells ( Fig. 6e ), while expressions of other hypoxia-inducible genes ( Phd3 , Serpine1 , Aldoc and Pfkfb3 ) ( [45] , [48] ) were not enriched in the ON-REP fraction ( Supplementary Fig. S13b ). These results imply that there are distinct hypoxic thresholds for the hypoxic gene transcription in REP cells. Two important regulatory elements, that is, the GATA site [14] and the liver-specific enhancer (EpoE-3′), have been identified in the Epo gene proximal region [5] , [9] . In this study, we have integrated these two elements within the 3.3-Epo3 ′ transgene into the Epo knockout mouse and rescued the mouse from embryonic lethality. The regulatory regions are sufficient to induce Epo expression in the liver, but insufficient to recapitulate renal Epo expression. Therefore, we have expected that the rescued mice would develop Epo-deficiency anaemia in adults. Expression profiles of the 3.3-Epo3 ′ transgene appeared to be affected by chromosomal integration sites, and the majority of the rescued mouse lines suffered from polycythaemia due to ectopic transgene expression. However, mice rescued by line-458 uniquely showed severe anaemia, and we established ISAM as a novel mouse model for postnatal Epo-deficiency anaemia, utilizing this line of mice. ISAM are fertile and the phenotype is stably transmitted through generations. ISAM shows typical characteristics of Epo-dependent renal anaemia. Compared with other mouse models of renal anaemia [15] , [25] , [26] , [49] , [50] , ISAM is unique as it genetically develops adult-onset anaemia without any treatments and the phenotype solely depends on the Epo-deficiency. ISAM provides advanced experimental means for investigation of Epo function in adulthood. Early erythroblasts are markedly impaired in the bone marrow of ISAM, and gene expression in the erythroblasts compared with other haematopoietic lineage cells are quickly altered by Epo administration into ISAM, indicating that erythroblasts are the main target of Epo signalling [5] , [33] , [51] and Epo is principally an erythroid growth factor [52] . Recent studies have shown pleiotropic functions for Epo, such as neuroprotection, cardioprotection, angiogenesis and inflammation [20] , [21] , [53] . Although we have observed no direct evidence for the non-erythropoietic functions of Epo in ISAM by brief observation, detailed analyses of this Epo-deficiency model may provide information on Epo function beyond erythropoiesis. The rHuEPO has been used widely as a powerful drug for anaemic patients [20] , [21] , [22] , but its downstream target genes are largely unknown. In this regard, previous studies mainly used primary culture systems for global gene expression analyses in which the erythroid precursors were stimulated with Epo [34] , [35] . Our in vivo microarray analysis employing ISAM revealed the Epo-responsive genes rapidly induced in the bone marrow as a result of Epo-deficient conditions. We found the Mmp13 gene encoding collagenase-3 to be an indirect downstream target of Epo signalling in addition to the known Epo-regulated genes. As this enzyme is produced by osteoblasts and chondrocytes for bone remodelling [39] , Epo is suggested to modulate the bone space for erythroid expansion, consistent with previous reports that Epo regulates skeletal homoeostasis and bone marrow microenvironment [34] , [40] . REP cells sense the hypoxic environmental signal and regulate Epo expression with an on-off mode [14] , [18] . Our GFP reporter mouse systems have enabled the identification and isolation of REP cells as peritubular fibroblastic cells with a neural cell phenotype [6] , [14] , [17] . The present study supports this previous finding, because isolated REP cells express the neural isoforms of glycolysis genes, such as Glut3 , Eno2 , Aldoc and Pfkfb3 genes. The number of identified REP cells is limited even under severe anaemic/hypoxic stress [14] , [18] , [19] . In this study, GFP expression enhanced by severe chronic anaemia in ISAM facilitated REP cell labelling under genetically reproducible conditions. The labelling efficiency was further improved by combination with the Cre- lox P system in Epo-Cre::R26T mice, such that cells that had activated the Epo gene locus were permanently labelled with tdTomato expression. It has been considered that renal Epo production is limited to a specific subset of peritubular interstitium [18] , [54] . Based on our results, together with the recent finding that REP cells and renal interstitial fibroblasts originate from the same lineage [41] , we propose that the Epo-producing potential is an innate property of whole interstitial fibroblasts distributed in the cortex and outer medulla. Therefore, a small fraction of REP cells are working as Epo-suppliers under certain anaemic/hypoxic conditions, while the vast majority of REP cells are resting. A threshold of hypoxia and/or other unidentified differences may define the two states involved in molecular mechanisms underlying hypoxia-inducible Epo gene regulation in REP cells. Additionally, ISAM is available to elucidate the roles of REP cells beyond the secretion of Epo, for example, examination of dynamic phenotypic changes of REP cells in injured kidneys. In conclusion, our results demonstrate that ISAM faithfully recapitulates nearly all aspects of Epo-deficiency anaemia. Additional analyses should provide further insight into how Epo-deficiency affects adult erythropoiesis and related complications without secondary effects of uraemic toxins and inflammatory cytokines, which often accumulate in renal anaemia patients. ISAM serves as a valuable experimental animal model to validate rHuEPO or ESAs and offers a promising monitoring system for REP cells in physiology and disease. Generation of transgene constructs To construct the 3.3 K-Epo3 ′ transgene, the Epo gene fragment between Cla I and Bam HI sites (3.3-kb upstream and 4.5-kb downstream from the transcriptional initiation site, respectively) was isolated from the 129/Sv mouse genome [5] and cloned into pBluescript II (Agilent Technologies). A 310-bp (base-pair) sequence in the 3′-untranslated region was removed by Eco RI digestion and self-ligation ( Fig. 1a ). For the Epo-Cre transgene construct, exons II–IV of the Epo gene in a BAC clone ( Epo-60 K/BAC ) were replaced with Cre cDNA (from pBS185, Gibco) by homologous recombination [14] at the same position with GFP cDNA placed in the Epo knockout allele. Mutation of the start codon was also introduced in the first exon to initiate translation from the start codon of Cre cDNA. The recombinant BAC clone was confirmed by digestion and sequencing, and purified as circular BAC DNA by ultra centrifugation with caesium chloride [55] . Gene-modified mouse lines Linearized 3.3 K-Epo3 ′ and circular Epo-Cre transgene constructs were microinjected into fertilized eggs from BDF1 mice (CLEA Japan). Eleven and three lines of 3.3 K-Epo3 ′ and Epo-Cre transgenic mice were established, respectively. The Epo knockout mouse line, in which GFP cDNA was knocked-in, has been described [6] . The Rosa26R-STOP-tdTomato mouse line [44] was obtained from Jackson Laboratory (Stock no. 007908). Genomic tail DNA was recovered from pups, and the Epo knockout allele and transgenes were detected by PCR genotyping. The wild-type Epo allele was discriminated from the knockout allele and transgenes, which were derived from the 129/Sv genome, using primers corresponding to the C57BL/6-specific sequence within the 3′-untranslated region. To determine the copy number of the transgene, qPCR of genomic DNA was performed using ABI7300 (Applied Biosystems) and SYBR Green reagent (Eurogentec, Seraing, Belgium). Sequence information on all primers used in the genotyping and copy number analysis is listed in Supplementary Table S1 . All mice were kept strictly in specific pathogen-free conditions, and were treated according to the regulations of The Standards for Human Care and Use of Laboratory Animals of the Tohoku University . Blood analysis and phlebotomy Mouse peripheral blood samples taken from the retro-orbital plexus or submandibular vein [56] were analysed by automatic cell counter (Nihon-Kohden, Tokyo). Peripheral blood smears were stained with Wright-Giemsa for morphological observation or new methylene blue for reticulocyte count. The acute anaemic condition was induced by phlebotomy taking 0.4 ml of peripheral blood at 48, 24 and 6 h before analysis. Plasma Epo concentrations were measured by Mouse Epo ELISA kit (R&D systems). Quantitative reverse transcription PCR Tissue total RNA was extracted using ISOGEN (Nippon-Gene), and cDNA was synthesized by Superscript III, RNase OUT and random primers (Invitrogen). qPCR of reverse-transcribed samples (RT–qPCR) was performed with target-specific primers using ABI7300. The expression level of 18S rRNA was used as an internal standard, and normalized values of Epo and GFP mRNA expressions were exhibited when a standard sample (mixture of kidney cDNAs from anaemic Epo +/– mice) was set as 100. The transgenic and endogenous Epo mRNA expressions were distinguished by semi-quantitative RT–PCR analysis using HPRT mRNA expression as an internal control. Sequence information for all primers used in the RT–PCR analysis is listed in Supplementary Table S2 . Flow cytometry For analyses of erythroid cells, single-cell suspensions from haematopoietic tissues were stained for 30 min with fluorescein isothiocyanate (FITC)-conjugated anti-CD71, phycoerythrin (PE)-conjugated anti-Ter119, allophycocyanin-conjugated anti-c-Kit, FITC-conjugated anti-Gr1, FITC-conjugated anti-Mac1, PE-conjugated anti-B220 and/or allophycocyanin-conjugated anti-CD3e antibodies (BD Pharmingen). To obtain cell suspensions containing REP cells, kidneys were minced and enzymatically digested with Liberase TM (0.26 U ml −1 , Roche) for 2 h at 37 °C in a shaking bath, followed by filtration using a 35-μm cell strainer. After staining dead cells with propidium iodide, flow cytometry was performed with fluorescence-activated cell sorting (FACS) Canto II, FACS Aria II and FACS Diva software (Becton Dickinson). Histological analysis Paraffin-embedded tissue sections (5-μm thickness), which were fixed in Mildform reagent (Wako), were stained by haematoxylin-eosin. For immunofluorescent staining, tissues were fixed in 4% paraformaldehyde for 2 h at 4 °C and embedded in OCT compound (Sakura Finetek Japan). Frozen sections (20-μm thickness) were incubated with chicken anti-GFP polyclonal antibody (1:500, ab13970, Abcam), rat anti-CD73 antibody (1:500, 12-0731-82, eBioscience), rat anti-PDGFRβ antibody (1:100, ab32570, Abcam) and/or biotinylated Lotus Tetragonolobus Lectin (1:50, B-1325, Vector labs) at 4 °C overnight. After washing, sections were incubated with Alexa Fluor 488-conjugated anti-chicken IgG (1:500, A-11039, Molecular Probes) and Alexa Fluor 555-conjugated anti-rat IgG antibodies (1:500, A-21434, Molecular Probes) and Alexa Fluor 350-conjugated streptavidin (1:100, S-11249, Molecular Probes) at room temperature for 1 h. Fluorescent images were obtained using the LSM510 confocal imaging system (Carl Zeiss). Administration of Epo antibody and recombinant Epo To neutralize Epo activities in mice, 200 μg of anti-mouse Epo or isotype monoclonal antibody (R&D systems) was injected into the intraperitoneal cavity every other day for 12 days. For Epo administration, rHuEPO (kind gift from Chugai Pharmaceutical, 3,000 U kg –1 body weight) was intraperitoneally injected every other day for 12 days. Microarray analysis Total RNA purified from mouse bone marrow was processed and hybridized to whole-mouse genome microarrays (4 × 44 K, Agilent Technologies) following the manufacturer’s procedure. The data were analysed with GeneSpring software (Silicon Genetics). Heat map analysis was performed as previously described [57] . Primary osteoblasts Osteoblast progenitors were prepared from neonatal (3−5 days old) mouse calvariae that were sequentially digested with 0.1% collagenase (Worthington Biochemical Corporation) in αminimum essential medium (Sigma). The cells expanded in αminimum essential medium containing 10% fetal bovine serum for 2 days were differentiated into osteoblasts by supplementation of β-glycerophosphate (10 mM), dexamethasone (0.1 μM) and ascorbate (50 μg ml –1 ) for a week [58] . Alkaline phosphatase staining (AP staining kit, Stemgent) confirmed that the purity of mature osteoblasts was >70%. Total RNA was isolated from the differentiated osteoblasts incubated for 24 h with or without rHuEPO (10 U ml −1 ). Statistical analysis All quantitative data were represented as the means with s.d. values. A two-sided, unpaired Student’s t -test was used for analyses of differences between groups. Statistical significance was considered as P <0.05. Accession code : Microarray data have been deposited in Gene Expression Omnibus database under accession code GSE43585 . How to cite this article: Yamazaki, S. et al . A mouse model of adult-onset anaemia due to erythropoietin deficiency. Nat. Commun. 4:1950 doi: 10.1038/ncomms2950 (2013).